Competition–colonization dynamics in experimental bacterial metacommunities One of the simplest hypotheses used to explain species coexistence is the competition–colonization trade-off, that is, species can stably coexist in a landscape if they show a trade-off between competitive and colonization abilities. Despite extensive theory, the dynamics predicted to result from competition–colonization trade-offs are largely untested. Landscape change, such as habitat destruction, is thought to greatly influence coexistence under competition–colonization dynamics, although there is no formal test of this prediction. Here we present the first illustration of competition–colonization dynamics that fully transposes theory into a controlled experimental metacommunity of two Pseudomonas bacterial strains. The competition–colonization dynamics were achieved by directly manipulating trade-off strength and colonization rates to generate the full range of coexistence conditions and responses to habitat destruction. Our study successfully generates competition–colonization dynamics matching theoretical predictions, and our results further reveal a negative relationship between diversity and productivity when scaling up to entire metacommunities. Competition–colonization (CC) trade-off models predict that species can coexist in landscapes with patch turnover by means of spatial niche partitioning [1] , [2] , [3] , [4] . Under CC dynamics, species can occupy a ‘colonization niche’ by efficiently colonizing empty habitat patches (that is, ‘fugitive species’) or a ‘competition niche’ by outcompeting other species within sites [5] . Depending on allocation trade-offs, such as those determined by life history, these alternative strategies (that is, ‘colonizers’ versus ‘competitors’) reduce the ratio of interspecific to intraspecific competition and allow coexistence to occur without environmental heterogeneity among patches [6] . Although early CC models [1] , [2] somewhat unrealistically assumed strict trade-offs, including habitat homogeneity and the absence of both patch pre-emption and stochasticity, CC model predictions have been shown to be applicable to situations of greater complexity [4] , [7] . CC models predict that changes to landscape structure impact coexistence even in the absence of changes in environmental conditions at the local scale [8] . A key prediction of such models is that habitat destruction (or any other environmental change that reduces overall colonization rates) should preferentially suppress superior competitors or drive them extinct, whereas increasing the regional abundance of inferior competitors [8] . If these landscape-level processes are resolved on long time scales, then extinction debts (that is, species committed to extinction) are expected to develop [9] . It is also likely that changes in the prevalence of competitively dominant species could alter ecosystem functioning if such species are more productive than inferior competitors [5] . Despite a general acceptance of the theoretical framework, to our knowledge there is no direct experimental treatment of the general predictions of the CC theory; in fact, indirect tests that attempted to document the existence of the CC trade-off have produced contradictory results in experimental [10] , [11] , [12] , [13] and observational studies of natural species assemblages [14] , [15] , [16] , [17] , [18] . Moreover, because the existence of a CC trade-off in an assemblage does not necessarily indicate that CC dynamics are determinant, indirect approaches have limited power to evaluate the theory. In this study, we present the first experimental illustration of a CC dynamic by manipulating the trade-off strength and colonization rate in an experimental system of Pseudomonas fluorescens bacteria in 96-well plate metacommunities. Pseudomonas has emerged as a model for experimental ecology and evolution [19] , [20] , [21] . We first tailored the general CC model [2] , [3] to our experimental system, which allowed us to make quantitative predictions regarding the conditions under which different patterns of coexistence and dominance are predicted in the metacommunity. We constructed and manipulated the two key mechanisms of CC dynamics in the model (trade-off strength and colonization rate) within a controlled setting to impose an experimental CC dynamic. We subsequently tested the predicted consequences of this dynamic for coexistence, landscape change and ecosystem function by monitoring strain persistence, local dominance, patch occupancy and metacommunity productivity. Our experiment is thus a targeted test of CC dynamics; however, it is an implementation rather than a test of underlying mechanisms. Experimental system We used two Pseudomonas bacterial strains (analogous to ecological species [22] ), a strong competitor (‘competitor’) and a poor competitor (‘colonizer’), to generate a strict asymmetry of competition in local patches (that is, the colonizer is completely excluded from local patches). The rationale underlying the use of a two-strain system is consistent with other existing experimental and empirical studies of the CC (for example, [13] , [15] , [18] ) and a variety of other studies that use microbes to investigate ecological phenomenon (for example, [23] , [24] , [25] ). We manipulated the strength of the CC trade-off by controlling the colonization of the two strains independently; both strains could have the same colonization rate in the experiment (no trade-off treatment) or the colonization rate of the colonizer could be strongly increased relative to the competitor (strong trade-off treatment). The manipulation of colonization rate was achieved by diluting each strain when building the ‘colonizers pool’ (when inoculating a new microplate between two time steps of our experiment); greater dilution reduced the number of cells that entered the colonizers pool and consequently reduced the probability that a strain would successfully colonize each inoculated well (see Methods and Supplementary Methods ). In contrast to most CC models that assume continuous colonization processes, we aimed to conduct our colonization treatments at discrete-time intervals for logistical feasibility. To achieve this goal, we needed to derive a discrete version of the CC competition model that we could parameterize for our experimental system (see Methods and Supplementary Methods ). The following experiments and model conditions were implemented. An initial metacommunity was inoculated with each of the two strains in half of the wells of a 96-well microplate. Every 24 h, the regional abundances (that is, microplate scale) of the two strains were estimated and used to build a ‘colonizer pool,’ which was subsequently used to inoculate a new microplate containing fresh medium. The relative contribution of the two strains in the colonizer pool and the dilution of this pool were adjusted before each transfer ( Fig. 1 ), to manipulate the absolute and relative colonization rates (and thus the strength of the CC trade-off) of the two strains in the metacommunity. This procedure ensured that our experimental manipulations remained constant throughout the experiment, but that potential deviations from the predicted trajectories in the preceding transfers would be taken into account in the computations of the colonization pool. The overall dilution ensured that colonization rates were low enough to approximate limited or near-limited dispersal and generate an exponential growth phase. To prevent any possible confounding of evolutionary changes in each strain from affecting the dynamics, at each new transfer, the bacterial colonization pool was reconstituted from initial frozen stock and not from the bacteria of the previous transfer. Using this experimental setting and our model ( Fig. 2 , see Methods ), we predicted the outcome of metacommunity dynamics under different trade-off and colonization scenarios ( Fig. 3 ). We subsequently assigned our primary experimental treatments along this parameter space to generate all predicted outcomes, which consisted of the exclusion of the colonizer or competitor, coexistence and the extinction of both strains ( Supplementary Table S1 ). In general, our experimental results closely corresponded to the predictions of our model. 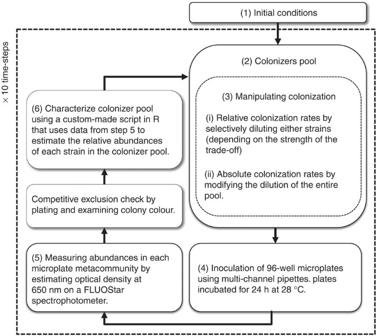Figure 1: Implementing competition–colonization trade-offs. The experiment consisted of six basic steps: (1) set up an initial metacommunity with equal proportions of both strains in all wells (48 wells at random occupied by each strain); (2) build a new ‘colonizer pool’ based on the regional abundances of the two strains after every 24 h; (3) modify the relative contribution of the two strains in the colonization pool and the dilution of this pool according to each experimental treatment (seeSupplementary Table 1) to manipulate the absolute and relative colonization rates (and thus the strength of the CC trade-off) of the two strains in the metacommunity; and finally (4) inoculate new metacommunities (that is, new microplates containing fresh media); (5) measuring abundances in each microplate metacommunity by estimating optical density; presence/absence results were confirmed via plating. Finally, (6) characterize colonizer pool using data from step 5 to estimate the relative abundances of each strain in the colonizer pool. This experimental procedure was run for ten transfers. Figure 1: Implementing competition–colonization trade-offs. The experiment consisted of six basic steps: (1) set up an initial metacommunity with equal proportions of both strains in all wells (48 wells at random occupied by each strain); (2) build a new ‘colonizer pool’ based on the regional abundances of the two strains after every 24 h; (3) modify the relative contribution of the two strains in the colonization pool and the dilution of this pool according to each experimental treatment (see Supplementary Table 1 ) to manipulate the absolute and relative colonization rates (and thus the strength of the CC trade-off) of the two strains in the metacommunity; and finally (4) inoculate new metacommunities (that is, new microplates containing fresh media); (5) measuring abundances in each microplate metacommunity by estimating optical density; presence/absence results were confirmed via plating. Finally, (6) characterize colonizer pool using data from step 5 to estimate the relative abundances of each strain in the colonizer pool. This experimental procedure was run for ten transfers. 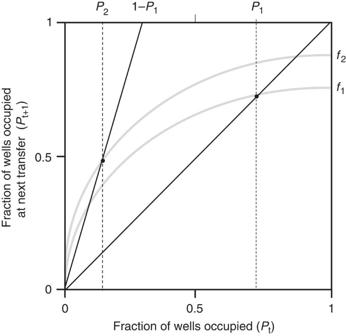Figure 2: Cobweb plot for the patch occupancy model. Patch occupancies after one transfer (P1for strain 1 andP2for strain 2 att+1) are functions of their current values through the probability of successful colonization following dispersal (f1andf2). The equilibrium is stable provided thatfis concave (f′′<0), and under this condition, the persistence conditions are f′1(0)>1 for strain 1 and f2′(0)>1/(1−P1) for strain 2. One can determine the equilibrium occupancy of the competitor (P1) and, subsequently, the equilibrium occupancy of the colonizer (P2), givenP1. Full size image Figure 2: Cobweb plot for the patch occupancy model. Patch occupancies after one transfer ( P 1 for strain 1 and P 2 for strain 2 at t +1) are functions of their current values through the probability of successful colonization following dispersal ( f 1 and f 2 ). The equilibrium is stable provided that f is concave ( f ′′<0), and under this condition, the persistence conditions are f′ 1 (0)>1 for strain 1 and f 2 ′(0)>1/(1− P 1 ) for strain 2. One can determine the equilibrium occupancy of the competitor ( P 1 ) and, subsequently, the equilibrium occupancy of the colonizer ( P 2 ), given P 1 . 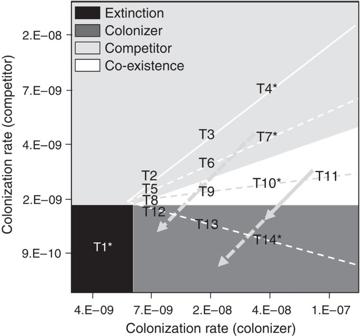Figure 3: Coexistence predictions. These predictions take into account the colonization rates (that is, dilution rates) of strong competitor (competitor) and poor competitor (colonizer) strains. Numbers indicate the treatment corresponding to each combination of strain colonization rates (obtained from the model presented inFig. 2). Axes indicate the colonization rates of the competitor and colonizer strains as the concentrations used before inoculation at each transfer; smaller values (that is, greater dilutions) indicate that fewer cells colonize each well (that is, are inoculated); greater values indicate more cells being dispersed. Light gray, colonizer excluded by the competitor; white, coexistence; dark gray, competitor excluded by the colonizer; black, extinction of both strains. Lines correspond to the four trade-off strengths: no trade-off (solid white line), weak, medium and strong trade-offs (all indicated by white dashed lines). Thicker arrows indicate the predicted trajectories of isolation treatments (H7 and H11) subjected to reductions in colonization rate (70 or 90%). *Treatments whose observed dynamics are displayed inFig 4. Dynamics for the remaining treatments are shown inSupplementary Fig. S1. Full size image Figure 3: Coexistence predictions. These predictions take into account the colonization rates (that is, dilution rates) of strong competitor (competitor) and poor competitor (colonizer) strains. Numbers indicate the treatment corresponding to each combination of strain colonization rates (obtained from the model presented in Fig. 2 ). Axes indicate the colonization rates of the competitor and colonizer strains as the concentrations used before inoculation at each transfer; smaller values (that is, greater dilutions) indicate that fewer cells colonize each well (that is, are inoculated); greater values indicate more cells being dispersed. Light gray, colonizer excluded by the competitor; white, coexistence; dark gray, competitor excluded by the colonizer; black, extinction of both strains. Lines correspond to the four trade-off strengths: no trade-off (solid white line), weak, medium and strong trade-offs (all indicated by white dashed lines). Thicker arrows indicate the predicted trajectories of isolation treatments (H7 and H11) subjected to reductions in colonization rate (70 or 90%). 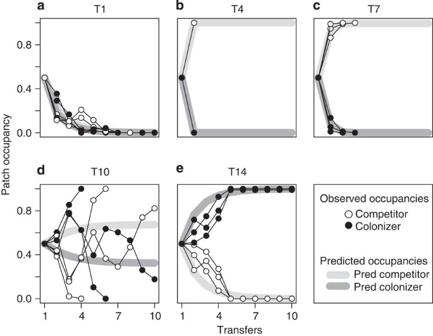Figure 4: Time series for all replicates from select treatments. Treatments T1, T4, T7, T10 and T14 are included. Panelsa–eshow observed occupancies (points) and model predictions for each strain (thick lines). Each treatment included three replicates and was run for a maximum of ten transfers. Replicates were stopped after the extinction of one or both strains occurred. Aside from treatment T10, which showed strong variability, all other treatments were consistent with the model predictions. Dynamics for the remaining treatments from the main experiment are shown in theSupplementary Fig. S1. *Treatments whose observed dynamics are displayed in Fig 4 . Dynamics for the remaining treatments are shown in Supplementary Fig. S1 . Full size image Coexistence and patch occupancy The persistence of both strains was most prevalent and resulted in the most even relative patch occupancies at moderate trade-off strength ( Figs 4 and Fig. 5 , and also see Supplementary Fig. S1 ). Treatments with no or weak trade-off strength resulted in the rapid exclusion of the colonizer, whereas strong trade-offs caused extinction of the competitor. Low absolute colonization resulted in the extinction of both strains. There was a highly significant interaction between strain identity and trade-off strength in predicting equilibrium patch occupancy ( Fig. 5 ; generalized-linear model, P <0.0001, df =74, χ 2 =32.81, Supplementary Table S2 ), which occurs because the two strains are affected in opposite ways by trade-off strength. Our experimental results thus showed that CC dynamics may regulate the outcome of species competition in a landscape that conforms to theoretical assumptions of strictly asymmetric competition, patch homogeneity and discrete global dispersal. Interestingly, the most important deviation between our predictions and the experimental results occurred under conditions for which our model predicted coexistence ( Supplementary Fig. S2 ). In half of such cases, either the competitor or the colonizer went extinct (four colonizer and two competitor extinctions). This evidence suggests that stochasticity may be important in CC dynamics, because it can lead to apparently random extinctions of either species, even under conditions that are favourable to the persistence of both strains. Our simulations indicate that these effects are not solely due to the finite size of the metacommunity [13] or to demographic stochasticity ( Supplementary Fig. S2 ), and that they are influenced by temporal variation (among transfers) in the overall colonization rates of the two species. In our experiments, this situation occurs because the actual colonization rates that we impose are highly sensitive to (1) density estimates in our metacommunities and stock cultures, (2) unavoidable procedural imprecision during dilution and (3) variability in the number of colonizing cells per well. This effect is likely to be comparable to the temporal stochasticity in overall dispersal that may occur in natural metacommunities. Figure 4: Time series for all replicates from select treatments. Treatments T1, T4, T7, T10 and T14 are included. Panels a – e show observed occupancies (points) and model predictions for each strain (thick lines). Each treatment included three replicates and was run for a maximum of ten transfers. Replicates were stopped after the extinction of one or both strains occurred. Aside from treatment T10, which showed strong variability, all other treatments were consistent with the model predictions. Dynamics for the remaining treatments from the main experiment are shown in the Supplementary Fig. S1 . 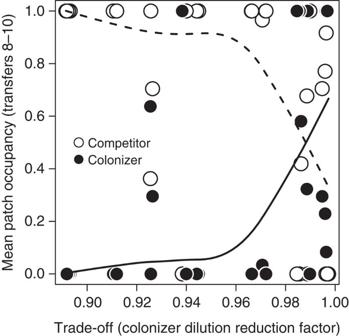Figure 5: Effect of trade-off strength on equilibrium patch occupancy by strain. Each point indicates the average proportion of occupied patches by each strain in each replicate (averages of transfers eight to ten in our experiment). The ‘competitor dilution reduction factor’ represents the proportional reduction in the overnight culture volume of the competitor before dilution (the strength of the trade-off in terms of reduced colonization rate). Treatment T1 was not included in this analysis because the extinction of both strains was predicted. A smoothing loess line is fitted to points from each strain to highlight the colonization pattern. All points were jittered to avoid overlap and improve the clarity of the figure. Full size image Figure 5: Effect of trade-off strength on equilibrium patch occupancy by strain. Each point indicates the average proportion of occupied patches by each strain in each replicate (averages of transfers eight to ten in our experiment). The ‘competitor dilution reduction factor’ represents the proportional reduction in the overnight culture volume of the competitor before dilution (the strength of the trade-off in terms of reduced colonization rate). Treatment T1 was not included in this analysis because the extinction of both strains was predicted. A smoothing loess line is fitted to points from each strain to highlight the colonization pattern. All points were jittered to avoid overlap and improve the clarity of the figure. Full size image Metacommunity productivity We found evidence for functional consequences of CC dynamics in a negative relationship between regional diversity and metacommunity productivity ( Fig. 6 ). Productivity was measured as the sum of cell densities (estimated by optical density) in all of the wells in each microplate averaged over the last three transfers. Taking in account that there were only two strains in this system, we calculated the Shannon index (or Shannon entropy) to measure diversity using the relative density of each strain within each microplate (that is, metacommunity). If both species were equally common, the Shannon index would be maximized. The more unequal the abundances of each strain are in the metacommunity, the smaller the corresponding Shannon index. If only one strain is contributing to the overall biomass and the other strain is very rare (or absent), the Shannon index approaches zero [26] . These scenarios are analogous to those in communities in which there are substantial changes in the relative proportions of abundant species, although not in numbers of species (for example, [27] , [28] ). In our experimental system, the competitor was much more productive (that is greater cell densities) than the colonizer ( Supplementary Fig. S3 ). Taking into account that these strains cannot coexist locally, the asymmetry in productivity implies that metacommunities dominated by the colonizer have lower productivity than those dominated by the competitor do. In fact, the low-diversity metacommunities often consisted of monocultures of the competitor with high productivity, whereas high-diversity metacommunities resulted in mixtures of productive (occupied by the competitor) and unproductive patches (occupied by the colonizer) that lead to a negative relationship between regional diversity and productivity ( Fig. 6 ). Theoretically, the low-diversity communities could also have consisted of monocultures of the colonizers, which would lead to a unimodal relationship between productivity and diversity [29] , but this scenario was not observed because there were far more treatments in which the competitor was expected to be more likely to persist than the colonizer ( Fig 3 ). 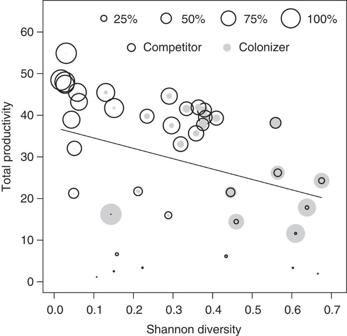Figure 6: Total metacommunity productivity and Shannon diversity. Points are averages from each replicate in the 14 main experimental treatments over transfers 8–10. Circle sizes are proportional to the mean patch occupancy of each strain (see scale in the figure). Notably, diversity was calculated based on the productivity and not the occupancy data, so plates with uneven occupancy can have high diversity (P<0.036,R2=0.108,F=0.57,n=42). Figure 6: Total metacommunity productivity and Shannon diversity. Points are averages from each replicate in the 14 main experimental treatments over transfers 8–10. Circle sizes are proportional to the mean patch occupancy of each strain (see scale in the figure). Notably, diversity was calculated based on the productivity and not the occupancy data, so plates with uneven occupancy can have high diversity ( P <0.036, R 2 =0.108, F =0.57, n =42). Full size image As opposed to other regional mechanisms of species coexistence that have found a positive biodiversity-ecosystem function (BEF; for example, source-sink dynamics [30] , [31] ), our experiment showed how CC dynamics may produce a rarely observed negative BEF relationship [32] , [33] , which is likely explained by a combination of patch dynamics and the regional dominance of a productive and competitive species (a ‘negative selection effect’, sensu [34] ). These results suggest that the definition of complementarity and selection effects, as the main drivers underlying the BEF relationship, may need to be revisited to accommodate broader coexistence mechanisms. Complementarity is based on niche differentiation and/or facilitation [35] , [36] and leads to a positive BEF, whereas the selection effect assumes that the dominant species are driving the BEF pattern and predicts either a positive or a negative relationship, depending on whether the traits of dominance are positively or negatively correlated to ecosystem functioning [34] . Although complementarity is clearly linked to the mechanism of species coexistence, the selection effect does not integrate any information on what drives species coexistence or abundances. In our experiment, dominance is linked to the proportion of patches occupied in the metacommunity and this is driven by an interaction between species traits (CC trade-off strength) and an external driver (perturbation rate) that ‘selects’ for dominance of either the competitor or colonizer. As dominance here is decoupled from species productivity (that is, the dominant species can be either the most or the least productive species), it leads to a negative selection effect where the most diverse metacommunities are less productive because they are dominated by the less productive species. Besides illustrating one of the first experimental negative BEF relationships (see also [32] , [37] ) our results stress the need for redefining the drivers of the BEF based on the relationship between the traits driving coexistence (for example, CC trade-offs versus local niche differentiation) and traits related to ecosystem functioning per se . Future research will need to disentangle the mechanisms driving species coexistence at local and regional scales, and reveal the manner in which niche traits at multiple scales are related to ecosystem functioning to advance a mechanistic understanding of the BEF relationship [29] , [38] , [39] . Increasing patch isolation In a second experiment, we investigated whether increased patch isolation could modify the outcome of metacommunity dynamics [8] , [9] . We reproduced two experimental treatments from the first experiment that revealed (1) the strong persistence of both strains and (2) rapid exclusion of the colonizer (treatments H11 and H7, respectively, in Fig. 7 ). We subsequently generated new predictions from the model, which showed that decreased overall colonization by 70 and 90% (corresponding to highly isolated patches) in each treatment ( Fig. 3 ) should qualitatively affect coexistence outcomes (eliminating the competitor from the H11 treatment, inducing coexistence in the H7 treatment). We ran these treatments in a second experiment with identical conditions for ten transfers. As predicted, we found that the persistence of both strains was enhanced for the 70% reduction and that the extinction of the best competitor (referred to as PI) was observed for the 90% reduction ( Fig. 7 ). Extinctions and reversals in persistence scenarios required multiple transfers to resolve relative to controls (especially in H7, Fig. 7 ), suggesting the existence of an ‘extinction debt’ [9] . This situation illustrates the susceptibility of communities structured by the CC trade-off to the changes in absolute colonization rate that are predicted under human impacts on landscapes, including habitat destruction [9] , [40] , fragmentation [8] or changes in inter-habitat matrix quality [41] . Previous experimental studies have been limited to binary or coarse-scale manipulations of colonization rate to simulate reductions in landscape connectivity [42] , [43] . By coupling our model predictions to a tailored experimental system, we were able to identify and test critical thresholds in the effects of decreased connectivity on metacommunities. Future developments will include measuring how these thresholds are affected by other scenarios of competitive interaction (for example, [4] ) or landscape topology and dispersal patterns (for example, [44] ). 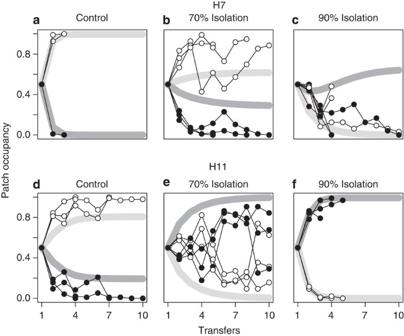Figure 7: Time series for all replicates from all treatments in the habitat isolation experiment. Panelsa–fshow observed occupancies (points) and model predictions for each strain (thick lines). Each treatment included three replicates and was run for a maximum of ten transfers. Replicates were stopped after the extinction of one or both strains occurred. Figure 7: Time series for all replicates from all treatments in the habitat isolation experiment. Panels a – f show observed occupancies (points) and model predictions for each strain (thick lines). Each treatment included three replicates and was run for a maximum of ten transfers. Replicates were stopped after the extinction of one or both strains occurred. Full size image In the context of increasing global change, ecologists are being urged to shorten the loop between theory and application [45] . Although ecologists have now adapted to include larger-scale mechanisms through the use of metapopulation, metacommunity and meta-ecosystem concepts and models [46] , [47] , [48] , [49] , experimental work targeting biodiversity and ecosystem effects at larger spatial scales is still in the initial stages [50] . The reality is that many theoretical models, often used to understand the consequences of global change, are difficult to test in natural systems, especially without first evaluating their performance in highly controlled experimental settings. Our study was done using a unitrophic community in an aquatic microcosm system, which is a common feature of many experimental tests of metacommunity paradigms [50] . These systems closely approximate theoretical assumptions and have a long history in ecology serving as bridges between theory and natural systems [51] , [52] , making them ideal for theory that is challenging to test like CC dynamics. Here we demonstrated that CC dynamics can indeed be implemented in a controlled microcosm system, facilitating the comprehensive and quantitative evaluation of these theoretical models in more robust situations. Our combined theoretical–experimental framework opens the way for further investigation of different aspects of CC dynamics (1) as a coexistence mechanism, (2) as a determinant of patterns of biodiversity loss under anthropogenic landscape impacts and (3) as a driver of regional BEF relationships. A prime example of the potential applications of our framework is the demonstration that the effects on landscape-level coexistence could be closely linked to those on regional level BEF relationships, suggesting that the effects of fragmentation on extinction debts may also cascade to ecosystem attributes. Our findings illustrate that BEF relationships may depend on the spatial scale over which they occur and the mechanisms generating the gradient of diversity [29] , [30] , [38] . We believe that our experimental framework is likely to prompt further investigations into the mechanisms underlying the evolution of CC dynamics in natural communities by exploring the particular ecological scenarios that trigger the evolution of CC trade-offs. As the changes in colonization rates in our experiment have analogous effects to reductions in the number of susceptible hosts or reduced transmissibility in epidemiological models [53] , [54] , our experimental setting has strong potential for use beyond community and landscape ecology questions; for example, to investigate questions related to spatial epidemiology. Our ability to bridge advances in theory with natural systems partially relies on using formal tests of predictions derived from theoretical models [51] , [52] . Although the highly controlled nature of our system and related experiments (for example, [55] , [56] ) does not allow direct extrapolation of our primary results to natural landscapes, they are a key step toward the understanding of natural metacommunity dynamics and properties. These approaches provide critical mechanistic explanations that will ultimately facilitate the application of theory towards the conservation and management of biodiversity and ecosystems on large scales. A model for CC dynamics in microplate metacommunities We used a patch occupancy model to describe how the proportion of wells (patches) in a microplate that are occupied by a particular bacterial strain changes through successive transfers from one plate to the next. This model can be seen as the discrete-time equivalent of seminal community ecology models [2] , [3] or the limiting case of a haystack metapopulation model when local competitive exclusion is rapid (see [57] ). With P 1 and P 2 as the proportion of wells occupied by strain 1 (competitor, equation 1) and strain 2 (colonizer, equation 2), respectively, the dynamic equations are as follows: where n 1 and n 2 are the local densities of each strain and d 1 and d 2 are their colonization rates; f is any function, including a Poisson zero-term function f = a (1− e (− bx )), such as the one used in this study. Important assumptions are that (1) strain 1 is completely dominant so that strain 2 disappears from any well where strain 1 is found; and (2) at the end of a transfer, both strains reach a given density in any colonized well, irrespective of initial conditions. The equilibrium occupancies can be determined graphically for any function f (see Fig. 2 ). Coexistence occurs if the proportion of successfully colonized wells exceeds zero for both strains and strain 2 has colonization rate sufficiently greater than strain 1 ( Fig. 3 ). We took dispersal to follow a Poisson distribution, which was appropriate for our method of diluting cell cultures [58] , and we assumed that at least one cell was needed for successful colonization, yielding f ( x )=1− e (− x ). This function was validated in preliminary trials ( Supplementary Fig. S4 ). Bacterial strains We used two isogenic strains for both experiments; Pseudomonas SBW25-LacZ (LacZ, ‘colonizer’) and an unknown strain of Pseudomonas were isolated on Gould S1 medium (sucrose, glycerol, casamino acids, NaHCO 3 , MgSO 4 7H 2 O, K 2 HPO 4 3H 2 O, N lauroyl sarcosine sodium, trimethoprim) from soil samples collected in Montpellier, France [59] . We refer to the second strain as ‘PI’ (‘competitor’). LacZ was chosen because it can be distinguished under plating with X-gal (5-bromo-4-chloro-3-indolyl-β- D -galactopyranoside) and IPTG (isopropyl-β- D -thio-galactoside). PI was chosen because it clearly outcompeted LacZ (see Supplementary Methods , Competitive assay section). In all trials and the main experiment, bacteria were grown for 24 h (overnight) at 28 °C on KB medium (glycerol 10 μl l −1 +20 g l −1 protease peptone H3+1.5 g l −1 K2HPO 4 +1.5 g l −1 MgSO 4 ; autoclaved 20 min at 121 °C) under constant agitation [21] . Model parameterization Preliminary trials showed that increasing the dilution rates generated a Poisson distribution of growth success in microplate wells ( Supplementary Fig. S4 ) and that this distribution was similar between the two strains. This result confirmed that we could manipulate colonization using pre-inoculation dilution and allowed us to use a specific distribution (Poisson) in our model. We parameterized our model with the average strain-specific growth in a single well after 24 h of 1.027 × 10 8 for LacZ and 9.517 × 10 8 cells for PI and the number of wells per microplate, which was 96. Colonization (dilution) rates were selected based on an exploration of model coexistence state outputs. Cell number was assayed following the droplet procedure described above. This model was implemented in Mathematica 8 (Wolfram). Model results are shown in Figs 3 , 4 and 7 . Basic experimental design The main experiment consisted of manipulating trade-off strength (that is, weak, moderate, strong and no trade-off) across 14 treatments ( Fig. 3 ), with 3 independent replicates for a starting total of 42 microplates (metacommunities), or 4,032 wells (patches). Our experiment consisted of six basic steps as follows: (1) set up an initial metacommunity with equal proportions of both strains in all wells (48 wells at random occupied by each strain); (2) build a new ‘colonizer pool’ based on the regional abundances of the two strains after every 24 h; (3) modify the relative contribution of the two strains in the colonization pool and the dilution of this pool according to each experimental treatment (see Fig. 1 ) to manipulate the absolute and relative colonization rates (and thus the strength of the CC trade-off) of the two strains in the metacommunity; and finally (4) inoculate new metacommunities (that is, new microplates containing fresh media); (5) measuring abundances in each microplate metacommunity by estimating optical density at 650 nm on a FLUOStar spectrophotometer; and (6) characterize colonizer pool using a custom-made script in R that uses data from step 5 to estimate the relative abundances of each strain in the colonizer pool (for complete description of these steps see Supplementary Methods , Detailed experimental protocol, and Supplementary Note for R script). This experimental procedure was run for 10 transfers, which we considered appropriate following model simulations ( Figs 4 and 7 ). The treatment- and strain-specific pre-inoculation dilution, concentrations of each strain and isolation levels can be found in Supplementary Table S1 . Similar to the main experiment, the isolation experiment had six basic steps as follows: (1) set up an initial metacommunity; (2) build a ‘colonizer pool’; (3) modify the relative contribution of the two strains in the colonizers pool and the dilution of this pool according to each experimental treatment and (4) inoculate new metacommunities. To mimic isolation, we imposed an additional reduction in overall colonization by reducing the inoculation volumes of the two strains by 0 (control), 70 or 90% in replicate microplates. The two coexistence scenarios that we implemented were the same as treatment T7 and T11 in the main experiment. Following the implementation of the additional reduction we proceeded with steps 5 and 6 as in the previous experiment. This experiment consisted of a starting total 18 microplates or 1,728 patches and was run for 10 transfers. Stock cultures and experimental duration A key issue in this experiment was to ensure that no substantial evolution occurred between transfers so as not to interfere with the ecological CC dynamics predicted by our model. For this purpose, we generated a uniform stock library of bacteria by freezing (−80 °C) 300 μl aliquots from overnight cultures in KB medium and glycerol (60/40 bacteria to glycerol, 80% v/v ratio). Before each transfer, we defrosted (for 5 min) and vortexed (for 10 s) new frozen aliquots to remove the glycerol from the aliquot before inoculation. Separate overnight tubes with 6 ml of KB were inoculated with 125 μl of LacZ and 30 μl of PI from the defrosted and vortexed aliquots. Previous pilot experiments have shown that these inoculation volumes ensured relative congruence between overnight growth and growth in the microplates. This detail meant that our procedure relating optical density-estimated cell counts in overnight cultures to microplate estimates (see Supplementary Methods , Measuring abundances and Detailed experimental protocol) was not correcting for great differences in cell counts. Overnight cultures were grown overnight at 28 °C under constant orbital shaking. Statistical analysis Productivity was measured as the sum of bacterial growth in all wells of each microplate. Diversity was calculated as the Shannon diversity index that takes into account the relative contribution to productivity of each strain. The Shannon index used was calculated as H =−Σ p i log( b ) p i , where p i is the proportional abundance of species i , and b is the base of the logarithm. This index is also known as Shannon entropy [26] . If both species are equally common, the Shannon index is maximized. The more unequal the abundances of each strain are in the metacommunity, the smaller the corresponding Shannon index. If only one strain is contributing to the overall biomass and the other strain is very rare (or absent), the Shannon index approaches zero [26] . These calculations were performed using the vegan package in R [60] . We tested for an interaction between strain identity and trade-off strength in predicting equilibrium patch occupancy using generalized-linear model ( Supplementary Table S2 ). How to cite this article: Livingston G. et al . Competition–colonization dynamics in experimental bacterial metacommunities. Nat. Commun. 3:1234 doi: 10.1038/ncomms2239 (2012).